Extracellular ATP mediates mast cell-dependent intestinal inflammation through P2X7 purinoceptors Mast cells are known effector cells in allergic and inflammatory diseases, but their precise roles in intestinal inflammation remain unknown. Here we show that activation of mast cells in intestinal inflammation is mediated by ATP-reactive P2X7 purinoceptors. We find an increase in the numbers of mast cells expressing P2X7 purinoceptors in the colons of mice with colitis and of patients with Crohn's disease. Treatment of mice with a P2X7 purinoceptor-specific antibody inhibits mast cell activation and subsequent intestinal inflammation. Similarly, intestinal inflammation is ameliorated in mast cell-deficient Kit W-sh/W-sh mice, and reconstitution with wild-type, but not P2x7 −/− mast cells results in susceptibility to inflammation. ATP-P2X7 purinoceptor-mediated activation of mast cells not only induces inflammatory cytokines, but also chemokines and leukotrienes, to recruit neutrophils and subsequently exacerbate intestinal inflammation. These findings reveal the role of P2X7 purinoceptor-mediated mast cell activation in both the initiation and exacerbation of intestinal inflammation. Both active and quiescent immunity occur simultaneously to achieve immunological homoeostasis in the harshest of environments—namely, the intestine. Aberrant immune responses in the gut lead to the development of intestinal immune diseases such as colitis and food allergies [1] , [2] . Mast cells (MCs) are generally recognized as major effector cells of type 1 allergic diseases, as well as of inflammation, host defenses, innate and adaptive immune responses and homoeostatic responses [3] , [4] , [5] . Histological analyses of patients with, and murine models of, colitis have implicated the involvement of MCs in intestinal inflammation [4] , [6] , but the factors responsible for MC activation are not fully understood. Several lines of evidence have demonstrated that release of extracellular ATP and ADP from injured, dying or activated cells acts as a danger signal by modulating various cellular functions via the activation of P2 purinoceptors [7] , [8] . P2 purinoceptors comprise P2X (P2X 1–7 ) and P2Y receptors (P2Y 1, 2, 4, 6, 11–14 ). P2X 1–7 receptors are ATP-gated ion channels and specific for ATP, whereas P2Y receptors are G protein-coupled receptors that are specific for ADP, UTP and ATP [7] , [8] . Stimulation by ATP or ADP through the P2 purinoceptors of macrophages and dendritic cells (DCs) results in the production of inflammatory cytokines; this can lead to the development of asthma, contact hypersensitivity or graft-versus-host disease [9] , [10] , [11] . MCs also express several P2 purinoceptors and release histamine, cytokines and chemokines upon nucleotide stimulation [12] . Although MCs are thought to be involved in intestinal inflammation, it is unclear whether extracellular nucleotides are required for this process. Here, we used a newly established anti-MC monoclonal antibody (mAb) to identify activated MCs and found that extracellular ATP mediates MC activation through P2X7 purinoceptors to initiate and amplify intestinal inflammation. Consequently, obstruction of the ATP-P2X7 purinoceptor cascade could be used to inhibit gut inflammatory diseases. Activated MCs in intestinal inflammation Using a 2,4,6-trinitrobenzene sulphonic acid (TNBS)-induced colitis model, we first examined whether MCs were involved in intestinal inflammation. To assess MC activation in vivo , we established an mAb (clone: 5A9) specific for CD63, a marker of activated MCs [13] . We confirmed that our anti-CD63 mAb was reactive specifically to MCs activated by immunoglobulin (Ig)E plus relevant allergen or a calcium ionophore, and not to naïve and CD63-knocked down MCs ( Supplementary Fig. S1 ). In the colons of TNBS-treated mice, increased numbers of CD63 + -activated MCs were noted until day 3 post administration; the numbers then gradually decreased and reached a basal level on day 6 ( Fig. 1a,b ), indicating that MC activation was associated with the initiation phase of colitis development, as previously reported in a murine model and in patients with inflammatory bowel disease [6] , [14] . It has generally been accepted that the mechanistic basis of ulcerative colitis (UC) and Crohn's disease (CD) are different. Indeed, the pathogenic cytokines involved in the development of UC and CD are different [2] and the genetic polymorphisms specific for UC and CD are also different [15] . In addition, the cytokines required for the development of MCs differ between humans (stem cell factor) and mice [interleukin (IL)-3 and stem cell factor] [4] . Thus, these different pathological environments may have led to differences in the requirement for, and involvement of, MCs in the development of inflammation. Therefore, we analysed MC numbers in both UD and CD patients, although we focused on the TNBS-induced colonic inflammation model. We detected increased numbers of MCs in the colons of patients with CD or UC ( Fig. 1c,d ). Thus, increased numbers of MCs in the colon is a characteristic of intestinal inflammation. 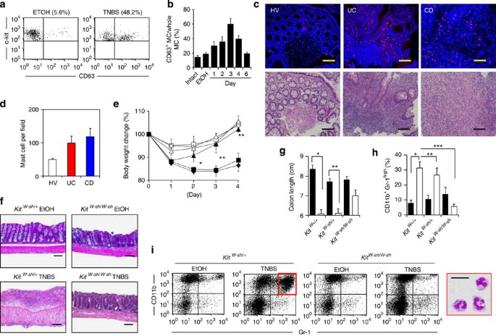Figure 1: Role of activated intestinal MCs in the development of intestinal inflammation. (a) CD63 expression on colonic MCs was examined with flow cytometry. Cells were gated on c-kit+and FcεRIα+cells. (b) The percentage of CD63+MCs in all c-kit+FcεRIα+MCs was determined with flow cytometry at various time points after TNBS administration (n=3 for day 6,n=5 for day 3,n=7 for intact, EtOH, day 1 and 2,n=14 for day 4). Control mice were analysed 4 days after EtOH administration (EtOH;n=7). Data are shown as means±s.e.m. (c) Colonic tissue sections from a healthy volunteer (HV) and UC and CD patients were stained with 4′,6-diamidino-2-phenyl indole (blue) and MC tryptase (red) or haematoxylin and eosin (H&E) (bottom). Scale bars, 100 μm. (d) Tryptase-positive MCs were counted in the fields of the tissue sections (four fields for each section). Data are means±s.e.m. (n=6). (e) Body weight changes were monitored after TNBS administration toKitW-sh/W-shMC-deficient mice (KitW-sh/W-shEtOH; open triangles:n=4,KitW-sh/W-shTNBS; closed triangles:n=9),Kit+/+control mice (Kit+/+EtOH; open diamonds:n=4,Kit+/+TNBS; closed diamonds:n=13) andKitW-sh/W+control mice (KitW-sh/W+EtOH; open squares:n=4,KitW-sh/W+TNBS; closed squares:n=11). Data are shown as percentages of baseline weights and are means±s.e.m., *P<0.0001 (two-tailed Student'st-test); **P=0.0024 (two-tailed Student'st-test). (f) The colon was isolated 4 days after TNBS treatment for H&E staining. Data are representative of at least three independent experiments. Scale bars, 100 μm. (g) Colon length was measured 4 days after colitis induction. EtOH, closed column; TNBS, open column. *P<0.0001 (two-tailed Student'st-test), **P=0.0024 (two-tailed Student'st-test). Data are shown as means±s.e.m. (h) The percentage of CD11b+Gr-1highcells in the colonic lamina propria was calculated, as measured with flow cytometry. EtOH, closed column; TNBS, open column. *P=0.0003 (two-tailed Student'st-test), **P=0.0029 (Welch'st-test) and ***P<0.0001 (Welch'st-test). Data are shown as means±s.e.m. (i) Colonic mononuclear cells were isolated 4 days after TNBS administration and stained with anti-CD11b and anti-Gr-1 antibodies. CD11b+Gr-1highcells were sorted and then stained with May-Giemsa stain. Scale bar, 20 μm. Data are representative of three experiments. Figure 1: Role of activated intestinal MCs in the development of intestinal inflammation. ( a ) CD63 expression on colonic MCs was examined with flow cytometry. Cells were gated on c-kit + and FcεRIα + cells. ( b ) The percentage of CD63 + MCs in all c-kit + FcεRIα + MCs was determined with flow cytometry at various time points after TNBS administration ( n =3 for day 6, n =5 for day 3, n =7 for intact, EtOH, day 1 and 2, n =14 for day 4). Control mice were analysed 4 days after EtOH administration (EtOH; n =7). Data are shown as means±s.e.m. ( c ) Colonic tissue sections from a healthy volunteer (HV) and UC and CD patients were stained with 4′,6-diamidino-2-phenyl indole (blue) and MC tryptase (red) or haematoxylin and eosin (H&E) (bottom). Scale bars, 100 μm. ( d ) Tryptase-positive MCs were counted in the fields of the tissue sections (four fields for each section). Data are means±s.e.m. ( n =6). ( e ) Body weight changes were monitored after TNBS administration to Kit W-sh/W-sh MC-deficient mice ( Kit W-sh/W-sh EtOH; open triangles: n =4, Kit W-sh/W-sh TNBS; closed triangles: n =9), Kit +/+ control mice ( Kit +/+ EtOH; open diamonds: n =4, Kit +/+ TNBS; closed diamonds: n =13) and Kit W-sh/W+ control mice ( Kit W-sh/W+ EtOH; open squares: n =4, Kit W-sh/W+ TNBS; closed squares: n =11). Data are shown as percentages of baseline weights and are means±s.e.m., * P <0.0001 (two-tailed Student's t -test); ** P =0.0024 (two-tailed Student's t -test). ( f ) The colon was isolated 4 days after TNBS treatment for H&E staining. Data are representative of at least three independent experiments. Scale bars, 100 μm. ( g ) Colon length was measured 4 days after colitis induction. EtOH, closed column; TNBS, open column. * P <0.0001 (two-tailed Student's t -test), ** P =0.0024 (two-tailed Student's t -test). Data are shown as means±s.e.m. ( h ) The percentage of CD11b + Gr-1 high cells in the colonic lamina propria was calculated, as measured with flow cytometry. EtOH, closed column; TNBS, open column. * P =0.0003 (two-tailed Student's t -test), ** P =0.0029 (Welch's t -test) and *** P <0.0001 (Welch's t -test). Data are shown as means±s.e.m. ( i ) Colonic mononuclear cells were isolated 4 days after TNBS administration and stained with anti-CD11b and anti-Gr-1 antibodies. CD11b + Gr-1 high cells were sorted and then stained with May-Giemsa stain. Scale bar, 20 μm. Data are representative of three experiments. Full size image To directly show the involvement of MCs in the development of intestinal inflammation, we used MC-deficient Kit W-sh/W-sh mice. We confirmed that immunological and inflammatory symptoms induced by TNBS treatment were identical in Kit W-sh/+ heterozygous and Kit +/+ homozygous mice; however, inflammatory symptoms, such as body weight loss, massive inflammatory cell infiltration and colon shortening, were restored in Kit W-sh/W-sh mice but not in Kit W-sh/+ heterozygous and Kit +/+ homozygous mice ( Fig. 1e–h ). Similarly, our histological and immunological analyses revealed that destruction of the colonic epithelial layer and infiltration by inflammatory cells—especially neutrophils, which were stained neutral pink and had lobulated nuclei,—were reduced in Kit W-sh/W-sh mice ( Fig. 1f,h,i ). Moreover, inflammatory signs were ameliorated in Kit W-sh/W-sh mice when we used other well-known inflammatory bowel disease models, such as the dextran sodium sulphate (DSS) colitis model ( Fig. 2a–c ). As the use of Kit W-sh/W-sh mice as an MC-deficient model is controversial [16] , [17] , we also used the MC-specific enhancer-mediated toxin receptor-mediated conditional cell knockout (TRECK) system (Mas-TRECK mice) [18] . We confirmed that specific depletion of MCs ameliorated the inflammation in this DSS-induced colitis model ( Fig. 2d–h ). Our data indicate that activated MCs participate in the aggravation of intestinal inflammation. 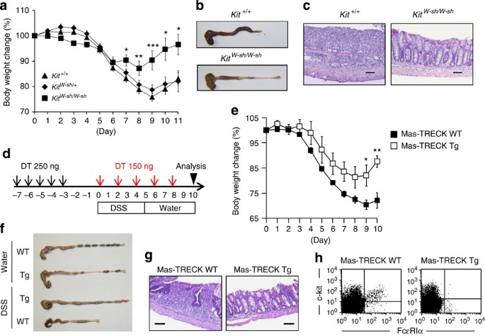Figure 2: Impaired DSS-induced colitis in MC-deficient mice. KitW-sh/W-shMC-deficient,Kit+/+control mice and Mas-TRECK transgenic (Tg) mice were subjected to DSS-induced colitis. (a) Body weight changes are shown as percentages of the baseline value and are means±s.e.m. (n=22 forKit+/+;n=25 forKitW-sh/+;n=10 forKitW-sh/W-sh). *P<0.01, **P=0.0207 and ***P=0.0004 (two-tailed Student'st-test). (b,c) Eleven days after DSS treatment, colon tissue and haematoxylin and eosin (H&E)-stained tissue sections were examined. Data are representative of at least three independent experiments. (d) Mas-TRECK Tg mice and their wild-type (WT) littermates were subjected to DSS-induced colitis. For diphtheria toxin (DT) treatment, mice were injected intraperitoneally with 250 ng of DT for 5 consecutive days (black arrows) and then with 150 ng every other day (red allows). (e) Body weight changes are shown as percentages of the baseline value and are means±s.e.m. (n=6 for Tg;n=10 for WT), *P=0.0107, **P=0.0037 (two-tailed Student'st-test). (f) Representative images of whole colons 10 days after DSS treatment. (g) Representative images of H&E staining. Scale bars, 100 μm. (h) Representative flow cytometric data of infiltrated c-kit+FcεRIα+MCs in the colon. Figure 2: Impaired DSS-induced colitis in MC-deficient mice. Kit W-sh/W-sh MC-deficient, Kit +/+ control mice and Mas-TRECK transgenic (Tg) mice were subjected to DSS-induced colitis. ( a ) Body weight changes are shown as percentages of the baseline value and are means±s.e.m. ( n =22 for Kit +/+ ; n =25 for Kit W-sh/+ ; n =10 for Kit W-sh/W-sh ). * P <0.01, ** P =0.0207 and *** P =0.0004 (two-tailed Student's t -test). ( b , c ) Eleven days after DSS treatment, colon tissue and haematoxylin and eosin (H&E)-stained tissue sections were examined. Data are representative of at least three independent experiments. ( d ) Mas-TRECK Tg mice and their wild-type (WT) littermates were subjected to DSS-induced colitis. For diphtheria toxin (DT) treatment, mice were injected intraperitoneally with 250 ng of DT for 5 consecutive days (black arrows) and then with 150 ng every other day (red allows). ( e ) Body weight changes are shown as percentages of the baseline value and are means±s.e.m. ( n =6 for Tg; n =10 for WT), * P =0.0107, ** P =0.0037 (two-tailed Student's t -test). ( f ) Representative images of whole colons 10 days after DSS treatment. ( g ) Representative images of H&E staining. Scale bars, 100 μm. ( h ) Representative flow cytometric data of infiltrated c-kit + FcεRIα + MCs in the colon. Full size image Establishment of an inhibitory MC-specific mAb IgE plus a relevant allergen induces MC activation; however, Rag-1 −/− and Tcrβ −/− δ −/− mice showed inflammatory responses comparable to those in TNBS-induced intestinal inflammation ( Supplementary Fig. S2a–d ) [19] and had increased numbers of CD63 + -activated MCs in their colons ( Supplementary Fig. S2e ), suggesting that T and B cells are not involved in MC activation during colitis. We also found no increase in CD63 expression on MCs after stimulation with IL-18 and IL-33, which are known to be involved in colitis ( Supplementary Fig. S2f ) [20] , [21] . We next tried to establish an anti-MC mAb that could ameliorate activated MC-mediated intestinal inflammation. We immunized rats with purified murine-activated colonic MCs, established hybridomas, performed flow cytometry to select hybridomas that produced mAbs that preferentially recognized colonic MCs and examined the hybridomas' ability to inhibit ovalbumin-induced food allergy [22] or TNBS-induced intestinal inflammation ( Supplementary Fig. S3 ). Among 2,000 clones, we obtained an anti-MC mAb (designated clone 1F11; rat IgG2b) that was strongly reactive to colonic MCs ( Fig. 3a ; Supplementary Fig. S3 ). In addition to colonic MCs, 1F11 mAb bound efficiently to peritoneal cavity-, lung- and bone marrow (BM)-derived MCs, but not to skin MCs ( Fig. 3a ). When tested with other immunocompetent cells in the colon, 1F11 mAb was weakly reactive to some CD3 + T cells, CD11c + DCs and F4/80 + macrophages, but was not reactive to Gr-1 + granulocytes, IgA + plasma cells or epithelial cells (ECs) ( Fig. 3b ). 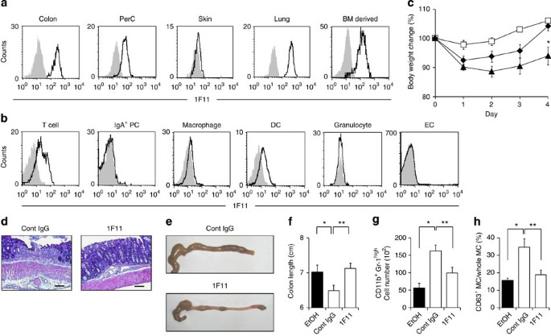Figure 3: Amelioration of colitis by treatment with intestinal MC-reactive 1F11 mAb. (a) MCs in the colonic lamina propria, peritoneal cavity (PerC), skin and lung, as well as BM-derived MCs, were stained with 1F11 mAb. Control staining with rat IgG2b is shown in grey. (b) Cells were isolated from colonic lamina propria and epithelium. CD3+T cells, IgA+plasma cells (PCs), F4/80+macrophages, CD11c+DCs, Gr1+granulocytes and ECs were gated and their reactivity to 1F11 mAb examined. Control staining with rat IgG2b is shown in grey. (c) C57BL/6 mice were treated with TNBS and their body weights were monitored for 4 days; 0.5 mg of 1F11 or the control mAb was intraperitoneally administered. Data from 9 (EtOH; open squares), 19 (TNBS with control mAb; closed triangles) and 12 (TNBS with 1F11 mAb; closed diamonds) mice. *P=0.0066 (Welch'st-test). Data are shown as percentages of baseline weights and are means±s.e.m. (d,e) Representative images of haematoxylin and eosin staining and colon tissue from 1F11 mAb-treated mice. Scale bars, 100 μm. (f) Colon length was measured 4 days after TNBS administration. *P=0.0445; **P=0.0073 (two-tailed Student'st-test). (g) Neutrophils (CD11b+Gr-1high) were quantified as percentages and numbers of cells. Data are shown as means±s.e.m. (n=6), *P<0.0001, **P=0.0047 (two-tailed Student'st-test). (h) Percentage of CD63+MCs in all c-kit+FcεRIα+MCs was determined with flow cytometry. Data are shown as means±s.e.m. (n=6) *P=0.0202; **P=0.0284 (two-tailed Student'st-test). Figure 3: Amelioration of colitis by treatment with intestinal MC-reactive 1F11 mAb. ( a ) MCs in the colonic lamina propria, peritoneal cavity (PerC), skin and lung, as well as BM-derived MCs, were stained with 1F11 mAb. Control staining with rat IgG2b is shown in grey. ( b ) Cells were isolated from colonic lamina propria and epithelium. CD3 + T cells, IgA + plasma cells (PCs), F4/80 + macrophages, CD11c + DCs, Gr1 + granulocytes and ECs were gated and their reactivity to 1F11 mAb examined. Control staining with rat IgG2b is shown in grey. ( c ) C57BL/6 mice were treated with TNBS and their body weights were monitored for 4 days; 0.5 mg of 1F11 or the control mAb was intraperitoneally administered. Data from 9 (EtOH; open squares), 19 (TNBS with control mAb; closed triangles) and 12 (TNBS with 1F11 mAb; closed diamonds) mice. * P =0.0066 (Welch's t -test). Data are shown as percentages of baseline weights and are means±s.e.m. ( d , e ) Representative images of haematoxylin and eosin staining and colon tissue from 1F11 mAb-treated mice. Scale bars, 100 μm. ( f ) Colon length was measured 4 days after TNBS administration. * P =0.0445; ** P =0.0073 (two-tailed Student's t -test). ( g ) Neutrophils (CD11b + Gr-1 high ) were quantified as percentages and numbers of cells. Data are shown as means±s.e.m. ( n =6), * P <0.0001, ** P =0.0047 (two-tailed Student's t -test). ( h ) Percentage of CD63 + MCs in all c-kit + FcεRIα + MCs was determined with flow cytometry. Data are shown as means±s.e.m. ( n =6) * P =0.0202; ** P =0.0284 (two-tailed Student's t -test). Full size image To show the inhibitory function of 1F11 mAb in intestinal inflammation, mice were given 1F11 mAb (0.5 mg day −1 in a single dose) for 3 days, beginning 1 day before intrarectal administration of TNBS. 1F11 mAb treatment reduced the intestinal inflammation ( Fig. 3c–g ) and decreased the number of CD63 + -activated MCs in 1F11 mAb-treated mice ( Fig. 3h ). Targeting P2X7 receptors reduces intestinal inflammation Mass spectrometry analyses of immunoprecipitants of MC cell lysates with 1F11 mAb showed that the P2X7 purinoceptor is recognized by 1F11 mAb ( Supplementary Fig. S4a ). The specificity of 1F11 mAb for the P2X7 purinoceptor was confirmed by its specific reactivity to cells transfected with P2X7 receptors but not with other types of P2X receptor (for example, P2X1 and P2X4; Supplementary Fig. S4b ). MCs derived from P2x7 −/− mice, however, were not recognized by 1F11 mAb ( Supplementary Fig. S4c ). Western blot and flow cytometric analysis showed that, among the several variants of P2X7 purinoceptors [23] , 1F11 mAb bound to variant a (full-length; Supplementary Fig. S4d,e ). In contrast, variant c (possessing the ATP-binding portion but lacking the C-terminal region) was detected by western blot, but its surface expression was not detected by flow cytometry because of its defect in extracellular expression ( Supplementary Fig. S4d,e ) [24] . In addition, neither western blot nor flow cytometry detected variant d (lacking the ATP-binding portion; Supplementary Fig. S4d,e ). These data strongly suggest that 1F11 mAb recognizes P2X7 receptors, specifically the ATP-binding portion. We also confirmed that 1F11 mAb had similar reactivity to that of a commercially available anti-P2X7 mAb (clone: Hano43; Supplementary Fig. S4f,g ). To evaluate whether 1F11 mAb directly affects MCs during ATP-mediated activation, we treated MCs with ATP in the presence of 1F11 mAb in vitro . 1F11 mAb treatment reduced the number of CD63 + -activated MCs induced by ATP in a dose-dependent manner ( Fig. 4a ). High concentrations of extracellular ATP increased the cell permeability of the MCs [12] . Thus, uptake of Lucifer yellow was observed in ATP-stimulated MCs but was substantially impaired in 1F11 mAb-treated and P2x7 −/− MCs ( Fig. 4b,c ). 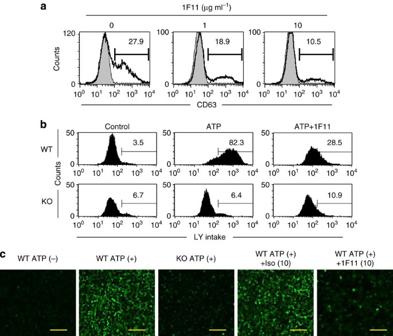Figure 4: Inhibition ofin vitroATP-mediated MC activation by 1F11 mAb. (a) BM-derived MCs, pretreated with various concentrations of 1F11 mAb (0, 1, 10 μg ml−1) for 15 min, were stimulated with 0.5 mM ATP for 30 min. Cells were stained with an anti-CD63 mAb for flow cytometric analysis. Data are representative of three independent experiments. (b) BM-derived MCs pretreated with various concentrations of 1F11 mAb or control rat IgG2b (0, 10 μg ml−1) for 15 min were stimulated with 0.5 mM ATP for 30 min in the presence of 1 mg ml-1Lucifer yellow (LY). (c) LY uptake was determined by using flow cytometry and fluorescence microscopy. Scale bar, 100 μm. Data are representative of three individual experiments. Figure 4: Inhibition of in vitro ATP-mediated MC activation by 1F11 mAb. ( a ) BM-derived MCs, pretreated with various concentrations of 1F11 mAb (0, 1, 10 μg ml −1 ) for 15 min, were stimulated with 0.5 mM ATP for 30 min. Cells were stained with an anti-CD63 mAb for flow cytometric analysis. Data are representative of three independent experiments. ( b ) BM-derived MCs pretreated with various concentrations of 1F11 mAb or control rat IgG2b (0, 10 μg ml −1 ) for 15 min were stimulated with 0.5 mM ATP for 30 min in the presence of 1 mg ml -1 Lucifer yellow (LY). ( c ) LY uptake was determined by using flow cytometry and fluorescence microscopy. Scale bar, 100 μm. Data are representative of three individual experiments. Full size image As many cell types (MCs, T cells and DCs) express P2X7 receptors ( Fig. 3b ), we then asked whether the P2X7 receptors on MCs were responsible for the MC-mediated intestinal inflammation in vivo by analysing MC-deficient Kit W-sh/W-sh mice reconstituted with P2x7 +/+ or P2x7 −/− MCs. We confirmed that reconstituted MCs were present in the colon and maintained P2X7 expression ( Supplementary Fig. S5 ). Like wild-type mice, Kit W-sh/W-sh mice reconstituted with P2x7 +/+ MCs showed severe inflammatory responses when treated with TNBS. However, these inflammatory responses were ameliorated when Kit W-sh/W-sh mice were reconstituted with P2x7 −/− MCs; the amelioration included inhibition of neutrophil infiltration and MC activation ( Figs 1 and 5a–f ). 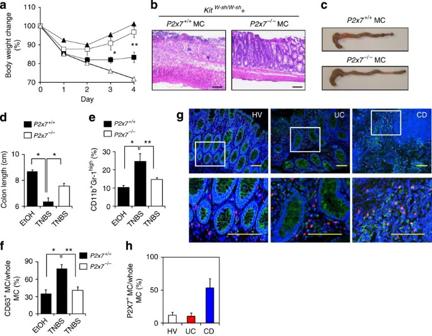Figure 5: Inhibitory targeting of P2X7 purinoceptors on MCs leads to amelioration of colonic inflammation. KitW-sh/W-shMC-deficient mice reconstituted withP2x7+/+,P2x7−/−orcaspase-1−/−BM-derived MCs were applied to a TNBS-induced colitis model. (a) Body weight changes were monitored in TNBS-treatedKitW-sh/W-shmice reconstituted withP2x7+/+(closed squares;n=9),P2x7−/−(open squares;n=7) orcaspase-1−/−(open triangles;n=4). BM-derived MCs were used for TNBS treatment, andP2x7+/+BM-derived MC-reconstitutedKitW-sh/W-shmice receiving EtOH served as controls (closed triangles;n=3). *P=0.0264 (two-tailed Student'st-test), **P=0.0058 (two-tailed Student'st-test). Data are shown as percentages of baseline weights and are means±s.e.m. (b) Representative images of haematoxylin and eosin staining are shown. Scale bars represents 100 μm. (c) Representative images of whole colons are shown. (d) Colon length was measured 4 days after TNBS administration. Data are shown as means±s.e.m. (n=3 forP2x7+/+EtOH,n=9 forP2x7+/+TNBS,n=7 forP2x7−/−TNBS), *P<0.001 (two-tailed Student'st-test). (e) Representative flow cytometric data of infiltrated neutrophils (CD11b+Gr-1high) in the colon from three individual experiments. *P=0.00741, **P=0.0009 (two-tailed Student'st-test). Data are shown as means±s.e.m. (f) The percentage of CD63+MCs in all c-kit+FcεRIα+MCs was determined with flow cytometry. Data are shown as means±s.e.m. (n=3–9), *P=0.007 (Welch'st-test), **P=0.0234 (Welch'st-test). (g) Colonic tissue sections from a healthy volunteer (HV) and from UC and CD patients were stained with 4′,6-diamidino-2-phenyl indole (blue), MC tryptase (red) and P2X7 (green). Scale bars, 100 μm. (h) Cells expressing both P2X7 and MC tryptase were counted in the fields of the tissue sections (four fields for each section). Data are means±s.e.m. (n=6). Figure 5: Inhibitory targeting of P2X7 purinoceptors on MCs leads to amelioration of colonic inflammation. Kit W-sh/W-sh MC-deficient mice reconstituted with P2x7 +/+ , P2x7 −/− or caspase-1 −/− BM-derived MCs were applied to a TNBS-induced colitis model. ( a ) Body weight changes were monitored in TNBS-treated Kit W-sh/W-sh mice reconstituted with P2x7 +/+ (closed squares; n =9), P2x7 −/− (open squares; n =7) or caspase-1 −/− (open triangles; n =4). BM-derived MCs were used for TNBS treatment, and P2x7 +/+ BM-derived MC-reconstituted Kit W-sh/W-sh mice receiving EtOH served as controls (closed triangles; n =3). * P =0.0264 (two-tailed Student's t -test), ** P =0.0058 (two-tailed Student's t -test). Data are shown as percentages of baseline weights and are means±s.e.m. ( b ) Representative images of haematoxylin and eosin staining are shown. Scale bars represents 100 μm. ( c ) Representative images of whole colons are shown. ( d ) Colon length was measured 4 days after TNBS administration. Data are shown as means±s.e.m. ( n =3 for P2x7 +/+ EtOH, n =9 for P2x7 +/+ TNBS, n =7 for P2x7 −/− TNBS), * P <0.001 (two-tailed Student's t -test). ( e ) Representative flow cytometric data of infiltrated neutrophils (CD11b + Gr-1 high ) in the colon from three individual experiments. * P =0.00741, ** P =0.0009 (two-tailed Student's t -test). Data are shown as means±s.e.m. ( f ) The percentage of CD63 + MCs in all c-kit + FcεRIα + MCs was determined with flow cytometry. Data are shown as means±s.e.m. ( n =3–9), * P =0.007 (Welch's t -test), ** P =0.0234 (Welch's t -test). ( g ) Colonic tissue sections from a healthy volunteer (HV) and from UC and CD patients were stained with 4′,6-diamidino-2-phenyl indole (blue), MC tryptase (red) and P2X7 (green). Scale bars, 100 μm. ( h ) Cells expressing both P2X7 and MC tryptase were counted in the fields of the tissue sections (four fields for each section). Data are means±s.e.m. ( n =6). Full size image We next analysed whether the MCs in UC or CD patients expressed P2X7. Although increased number of MCs were observed in the colons of both UC and CD patients ( Fig. 1c,d ), P2X7 purinoceptors were expressed by the MCs in CD patients but not by those in UC patients or healthy volunteers ( Fig. 5g,h ). Thus, it is likely that P2X7 purinoceptor-mediated MC activation also occurs in the human colon, especially in CD patients. To examine whether ATP was extracellularly released at high concentrations at inflammatory sites, we next measured ATP release from inflammatory colonic tissues. An elevated level of ATP release from the colon tissue was noted in TNBS-treated mice ( Fig. 6a ). In addition, intrarectal administration of non-hydrolyzable ATP (adenosine 5′- O -(3-thio) triphosphate and O -(4-benzoyl)benzoyl adenosine 5′-triphosphate) led to MC activation in the colonic tissue, similar to the effect of TNBS treatment ( Fig. 6b ). In contrast, intrarectal administration of other P2Y receptor agonists did not increase colonic MC activation ( Fig. 6b ). These findings indicate that inflammatory stimuli induce the extracellular release of ATP, which in turn leads to P2X7-dependent MC activation in the colon and subsequent exacerbation of intestinal inflammation. 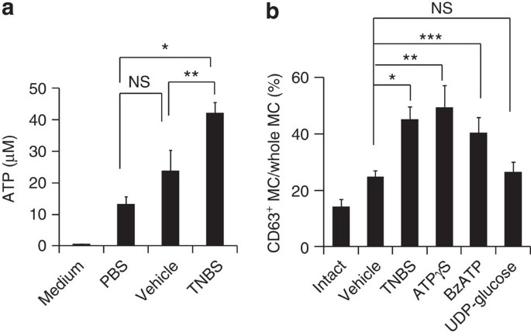Figure 6: Enhanced ATP production in intestinal inflammation and MC activation induced by non-hydrolyzable ATP. (a) The concentration of ATP released from the colon tissue of mice receiving intrarectally administered phosphate-buffered saline, vehicle or TNBS was measured. Data are shown as means±s.e.m. (n=3–7). *P=0.0004, **P=0.0447 (two-tailed Student'st-test). (b) CD63 expression of colonic MCs was measured with flow cytometry after intrarectal administration of vehicle (n=14), TNBS (n=5), non-hydrolyzable ATP (adenosine 5′-O-(3-thio) triphosphate (ATPγS);n=9 or O-(4-benzoyl)benzoyl adenosine 5′-triphosphate (BzATP);n=10) or UDP-glucose (n=6), or in intact mice (n=7). Data are shown as means±s.e.m. *P=0.0002 (two-tailed Student'st-test), **P=0.0135 (Welch'st-test) and ***P=0.0238 (Welch'st-test). NS, not significant. Figure 6: Enhanced ATP production in intestinal inflammation and MC activation induced by non-hydrolyzable ATP. ( a ) The concentration of ATP released from the colon tissue of mice receiving intrarectally administered phosphate-buffered saline, vehicle or TNBS was measured. Data are shown as means±s.e.m. ( n =3–7). * P =0.0004, ** P =0.0447 (two-tailed Student's t -test). ( b ) CD63 expression of colonic MCs was measured with flow cytometry after intrarectal administration of vehicle ( n =14), TNBS ( n =5), non-hydrolyzable ATP (adenosine 5′-O-(3-thio) triphosphate (ATPγS); n =9 or O-(4-benzoyl)benzoyl adenosine 5′-triphosphate (BzATP); n =10) or UDP-glucose ( n =6), or in intact mice ( n =7). Data are shown as means±s.e.m. * P =0.0002 (two-tailed Student's t -test), ** P =0.0135 (Welch's t -test) and *** P =0.0238 (Welch's t -test). NS, not significant. Full size image P2X7 signalling activates the caspase-1 inflammasome to induce the production of IL-1β and IL-18 (ref. 25 ). IL-1β production is also mediated by MC proteases, such as chymases [26] . We therefore examined whether MCs produced IL-1β via P2X7 receptor activation, and if so whether this production was caspase-1-dependent. IL-1β production was decreased when P2X7-deficient MCs were stimulated with ATP, whereas substantial amounts of IL-1β were produced in caspase-1-deficient MCs ( Supplementary Fig. S6 ), indicating that IL-1β production was P2X7-dependent but caspase-1-independent. In line with this finding, body weight changes were noted in Kit W-sh/W-sh mice reconstituted with caspase-1 −/− MCs ( Fig. 5a ). These results suggest that MC-dependent inflammation through P2X7 purinoceptors is not dependent on caspase-1-mediated IL-1β or IL-18 production. An autocrine loop of ATP conversion mediates MC activation In addition to ATP, other nucleotides (for example, extracellular ADP) act as signals to induce inflammatory responses [27] . We confirmed that MCs are activated by high concentrations of ADP and ATP ( Fig. 7a,b ). Extracellular ATP is hydrolysed by ectonucleoside triphosphate diphosphohydrolases (CD39) to ADP and AMP; it is then further hydrolysed by ecto-5′-nucleotidase (CD73) to adenosine, which has anti-inflammatory functions [27] . Colonic MCs expressed CD39 but not CD73 ( Supplementary Fig. S7a,b ), indicating that MCs can convert ATP to ADP but not to adenosine. We therefore examined the involvement of ADP-reactive P2Y purinoceptors and found that P2Y1 and P2Y12 were highly expressed on colonic MCs ( Fig. 7c ). However, inhibitors of P2Y1 and P2Y12 receptors, as well as knockdown of the P2Y12 receptor, had no effect on the induction of CD63 + -activated MCs ( Fig. 7d,e ; Supplementary Fig. S8a ). Similarly, intestinal inflammation, as well as activation of colonic MCs, was unaffected in clopidogrel (a P2Y12 receptor inhibitor)-treated mice ( Supplementary Fig. S8b–d ). These data indicate that although P2Y1 and P2Y12 were expressed on MCs neither P2Y1 nor P2Y12 purinoceptors mediate ADP-dependent CD63 + MC induction. 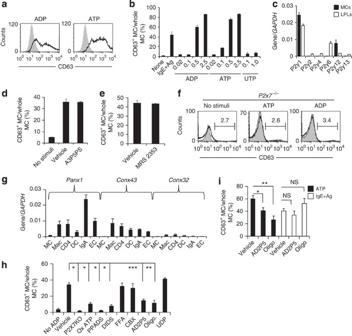Figure 7: The ecto-adenylate kinase pathway mediates ADP-dependent MC activation through P2X7 purinoceptors. (a) BM-derived MCs treated with ADP or ATP at 0.5 mM for 30 min and examined for CD63 expression. (b) BM-derived MCs treated with IgE plus relevant allergen or various concentrations of ADP, ATP or UTP for the analysis of CD63 expression. Data are representative of four experiments. (c) Expression of mRNA encoding each P2Y receptor in colonic lamina propria lymphocytes (LPLs) and MCs was analysed by quantitative reverse transcription (RT)–PCR (n=3). (d,e) BM-derived MCs pre-treated with 0.25 mM P2Y1 inhibitor (Adenosine-3-phosphate 5-phosphosulfate (A3P5PS)) (d) or 0.01 mM P2Y12 inhibitor (MRS2353) (e), stimulated with ADP and examined for CD63 expression (n=3). (f) BM-derived MCs fromP2x7−/−mice stimulated with ATP or ADP; CD63 expression was determined with flow cytometry. Data are representative of four experiments. (g) Expression of pannexin-1 (Panx1), connexin-43 (Conx43) and Conx32 on colonic MCs, macrophages (Mac), CD4+T cells (CD4), DCs, IgA+cells (IgA) and ECs was measured by quantitative RT–PCR (n=4). (h) BM-derived MCs were pretreated with inhibitors of P2X receptors [OxATP, 0.5 mM; pyridoxal-phosphate-6-azophenyl-2′,4′-disulfonate (PPADS); 4,4′-diisothiocyanatostilbene-2,2′-disulfonic acid (DIDS)], connexins [flufenamic acid (FFA)], Panx-1 [carbenoxolone (CBX)], ecto-adenylate kinase [diadenosine pentaphosphate (AD2P5)], ATP synthase (oligomycin) or nucleoside diphosphokinase (UDP) and subsequently stimulated with 0.25 mM ADP. CD63 expression was determined with flow cytometry. (n=3) *P<0.01, **P<0.05 (two-tailed Student'st-test). All data are shown as means±s.e.m. (i) BM-derived MCs were treated with AD2P5, oligomycin or UDP and stimulated with 0.5 mM ATP or IgE plus allergen. CD63 expression was determined with flow cytometry (n=5). *P<0.0001 (two-tailed Student'st-test), **P=0.0008 (two-tailed Student'st-test) and ***P=0.0008 (Welch'st-test). NS, not significant. Figure 7: The ecto-adenylate kinase pathway mediates ADP-dependent MC activation through P2X7 purinoceptors. ( a ) BM-derived MCs treated with ADP or ATP at 0.5 mM for 30 min and examined for CD63 expression. ( b ) BM-derived MCs treated with IgE plus relevant allergen or various concentrations of ADP, ATP or UTP for the analysis of CD63 expression. Data are representative of four experiments. ( c ) Expression of mRNA encoding each P2Y receptor in colonic lamina propria lymphocytes (LPLs) and MCs was analysed by quantitative reverse transcription (RT)–PCR ( n =3). ( d , e ) BM-derived MCs pre-treated with 0.25 mM P2Y1 inhibitor (Adenosine-3-phosphate 5-phosphosulfate (A3P5PS)) ( d ) or 0.01 mM P2Y12 inhibitor (MRS2353) ( e ), stimulated with ADP and examined for CD63 expression ( n =3). ( f ) BM-derived MCs from P2x7 −/− mice stimulated with ATP or ADP; CD63 expression was determined with flow cytometry. Data are representative of four experiments. ( g ) Expression of pannexin-1 (Panx1), connexin-43 (Conx43) and Conx32 on colonic MCs, macrophages (Mac), CD4 + T cells (CD4), DCs, IgA + cells (IgA) and ECs was measured by quantitative RT–PCR ( n =4). ( h ) BM-derived MCs were pretreated with inhibitors of P2X receptors [OxATP, 0.5 mM; pyridoxal-phosphate-6-azophenyl-2′,4′-disulfonate (PPADS); 4,4′-diisothiocyanatostilbene-2,2′-disulfonic acid (DIDS)], connexins [flufenamic acid (FFA)], Panx-1 [carbenoxolone (CBX)], ecto-adenylate kinase [diadenosine pentaphosphate (AD2P5)], ATP synthase (oligomycin) or nucleoside diphosphokinase (UDP) and subsequently stimulated with 0.25 mM ADP. CD63 expression was determined with flow cytometry. ( n =3) * P <0.01, ** P <0.05 (two-tailed Student's t -test). All data are shown as means±s.e.m. ( i ) BM-derived MCs were treated with AD2P5, oligomycin or UDP and stimulated with 0.5 mM ATP or IgE plus allergen. CD63 expression was determined with flow cytometry ( n =5). * P <0.0001 (two-tailed Student's t -test), ** P =0.0008 (two-tailed Student's t -test) and *** P =0.0008 (Welch's t -test). NS, not significant. Full size image It is generally accepted that P2X7 purinoceptors specifically recognize ATP [7] , but we found that they were also involved in ADP-mediated MC activation. Indeed, no activation was noted in P2x7 −/− MCs when they were stimulated with ADP ( Fig. 7f ), leading us to hypothesize that ADP promotes ATP release from MCs and their subsequent stimulation. To test this hypothesis, we measured the expression of pannexin-1, connexin 43 and connexin 32, which are ATP-releasing hemichannels, during cell activation [28] , [29] . The hemichannels were rarely expressed on the colonic MCs ( Fig. 7g ), and no inhibitory effect was observed when the MCs were treated with ADP in the presence of hemichannel inhibitors (flufenamic acid and carbenoxolone). However, cell activation was inhibited by P2X7 antagonists [oxidized ATP (OxATP), pyridoxal-phosphate-6-azophenyl-2′,4′-disulfonate and 4,4′-diisothiocyanatostilbene-2,2′-disulfonic acid disodium salt hydrate] ( Fig. 7h ). To further exclude the possibility that ADP triggers ATP release, we stimulated MCs with another P2Y ligand (UTP); we found that UTP did not induce MC activation ( Fig. 7b ). We then tested whether ADP was converted to ATP by ATP-converting enzymes such as ecto-adenylate kinase, ATP synthase and nucleoside diphosphokinase [30] . To test the involvement of these enzymes, we used inhibitors of ecto-adenylate kinase (diadenosine pentaphosphate; AD2P5), ATP synthase (oligomycin; oligo) and nucleoside diphosphokinase (UDP), and we found that inhibition of ecto-adenylate kinase and ATP synthase, but not nucleoside diphosphokinase, reduced ADP- as well as ATP-dependent MC activation ( Fig. 7h,i ). Neither AD2P5 nor oligo inhibited MC activation induced by the crosslinking of IgE with relevant allergen ( Fig. 7i ). Among the adenylate kinases, adenylate kinase 1 (AK1) and AK2 were expressed in colonic MCs, and the expression of AK2 was much higher than that of AK1 ( Supplementary Fig. S9a ). As with AD2P5 treatment, knockdown of AK2, but not AK1, led to the inhibition of both ADP- and ATP-mediated MC activation ( Supplementary Fig. S9b ). These results indicate that P2X7 purinoceptors have an important role in the activation of MCs by ATP, including ATP derived from ADP by the action of ecto-enzymes such as ATP synthase and AK2. Neutrophil infiltration by MC-derived mediators Evaluation of MC activation on the basis of CD63 expression is an important criterion [13] ; however, degranulation is not absolutely associated with cytokine production [31] . Therefore, we measured MC production of an array of inflammatory cytokine, chemokine and lipid mediators to additionally elucidate the role of P2X7 purinoceptor-mediated MC activation in the development of intestinal inflammation. Stimulation of MCs with ATP induced the production of inflammatory cytokines such as IL-6, tumour necrosis factor (TNF)α and oncostatin M [32] ; this induction was not observed in P2x7 −/− MCs or in wild-type MCs treated with 1F11 mAb ( Fig. 8a,b ). 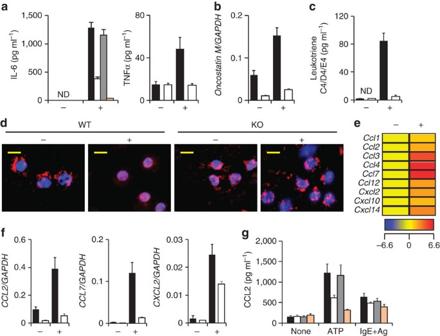Figure 8: Critical role of the intestinal MC-associated ATP-P2X7 purinoceptor pathway for induction of neutrophil infiltration. P2x7+/+andP2x7−/−BM-derived MCs were treated with 0.25 mM ATP (+) or left untreated (−). (a) Production of IL-6 (left panel; isotype mAb-treated MC, closed column; 1F11 mAb-treated MC, open column;P2x7+/+, grey column; andP2x7−/−, beige column) and TNFα (right panel) in culture supernatant (P2x7+/+, closed column;P2x7−/−, open column) was determined after 24 h stimulation. ND, not detected. Data are shown as means±s.e.m. (n=3). (b) Oncostatin M mRNA expression was measured 30 min after stimulation ofP2x7+/+(closed column) andP2x7−/−(open column) MCs with ATP. Data are shown as means±s.e.m. (n=3). (c) LT C4/D4/E4 production from ATP-stimulated (+) or -unstimulated (−)P2x7+/+(closed column) orP2x7−/−BM-derived MCs (open column) in culture supernatants was measured by using enzyme-linked immunosorbent assay (ELISA). Data are shown as means±s.e.m. (n=3). ND, not detected. (d)P2x7+/+andP2x7−/−BM-derived MCs were stimulated with 0.5 mM ATP. Cells were fixed and stained with an anti-5LO antibody (red) and 4′,6-diamidino-2-phenyl indole (blue). Scale bar, 10 μm. Data are representative of two experiments. (e) Representative data of a chemokine gene array are shown. Increased levels of each chemokine are shown as a heat map. (f) mRNA expression of CCL2 (left), CCL7 (middle) and CXCL2 (right) was measured by using quantitative reverse transcription–PCR. Data are shown as means±s.e.m. (n=3). (g) CCL2 production was enumerated by using ELISA 24 h after stimulation of BM-derived MCs with ATP or IgE plus antigen (IgE+Ag). Isotype mAb-treated MC, closed column; 1F11 mAb-treated MC, open column;P2x7+/+MC, grey column; andP2x7−/−MC, beige column). Data are shown as means±s.e.m. (n=3). Figure 8: Critical role of the intestinal MC-associated ATP-P2X7 purinoceptor pathway for induction of neutrophil infiltration. P2x7 +/+ and P2x7 −/− BM-derived MCs were treated with 0.25 mM ATP (+) or left untreated (−). ( a ) Production of IL-6 (left panel; isotype mAb-treated MC, closed column; 1F11 mAb-treated MC, open column; P2x7 +/+ , grey column; and P2x7 −/− , beige column) and TNFα (right panel) in culture supernatant ( P2x7 +/+ , closed column; P2x7 −/− , open column) was determined after 24 h stimulation. ND, not detected. Data are shown as means±s.e.m. ( n =3). ( b ) Oncostatin M mRNA expression was measured 30 min after stimulation of P2x7 +/+ (closed column) and P2x7 −/− (open column) MCs with ATP. Data are shown as means±s.e.m. ( n =3). ( c ) LT C4/D4/E4 production from ATP-stimulated (+) or -unstimulated (−) P2x7 +/+ (closed column) or P2x7 −/− BM-derived MCs (open column) in culture supernatants was measured by using enzyme-linked immunosorbent assay (ELISA). Data are shown as means±s.e.m. ( n =3). ND, not detected. ( d ) P2x7 +/+ and P2x7 −/− BM-derived MCs were stimulated with 0.5 mM ATP. Cells were fixed and stained with an anti-5LO antibody (red) and 4′,6-diamidino-2-phenyl indole (blue). Scale bar, 10 μm. Data are representative of two experiments. ( e ) Representative data of a chemokine gene array are shown. Increased levels of each chemokine are shown as a heat map. ( f ) mRNA expression of CCL2 (left), CCL7 (middle) and CXCL2 (right) was measured by using quantitative reverse transcription–PCR. Data are shown as means±s.e.m. ( n =3). ( g ) CCL2 production was enumerated by using ELISA 24 h after stimulation of BM-derived MCs with ATP or IgE plus antigen (IgE+Ag). Isotype mAb-treated MC, closed column; 1F11 mAb-treated MC, open column; P2x7 +/+ MC, grey column; and P2x7 −/− MC, beige column). Data are shown as means±s.e.m. ( n =3). Full size image We showed that neutrophil infiltration into the colon was mediated by MC activation ( Fig. 1h,i ), and a previous study suggested that neutrophil infiltration is a potential target in colitis treatment [33] . Consistent with these findings, ATP stimulation induced MCs, but not P2x7 −/− MCs, to produce leukotrienes (LTs; LT C4/D4/E4), which are associated with the translocation of 5-lipoxygenase (5-LO) into the nucleus—an important step for LT synthesis in MCs [34] ( Fig. 8c,d ). Also, chemokine gene array analysis demonstrated that ATP stimulation of MCs induced the expression of chemokines, including CCL2, CCL7 and CXCL2 ( Fig. 8e–g ), and 1F11 mAb treatment or P2X7 deficiency resulted in decreased CCL2 production from MCs activated by ATP but not by IgE plus allergen ( Fig. 8g ). Furthermore, Kit W-sh/W-sh mice showed decreased levels of both CCL2 and IL-1β in the colon tissue, but the production levels of these molecules recovered when the mice were reconstituted with wild-type MCs ( Supplementary Fig. S10a ). As neutrophils express the corresponding chemokine receptors, it is likely that ATP-dependent MC activation induced inflammatory neutrophil infiltration into the colon from the peripheral blood ( Supplementary Fig. S10b,c ), given the high level of TNFα production by the neutrophils ( Supplementary Fig. S10d ). These results indicate that ATP-dependent MC activation has key roles in the induction of inflammatory responses (by inducing inflammatory cytokines) and in the exacerbation of inflammatory responses (by inducing LTs and chemokines to recruit TNFα-producing neutrophils to the colon). Here, we showed that MCs have a critical role in the severity of colitis through their interaction with ATP and P2X7 purinoceptors. These interactions not only induce MC-mediated inflammatory responses but also exacerbate them by promoting neutrophil infiltration. Indeed, MC-deficient mice reconstitution with wild-type, but not P2x7 −/− , MCs resulted in neutrophil infiltration and severe inflammatory responses, together with increased production of IL-1β, LTs and CCL2 ( Figs 5 and 8 , and Supplementary Fig. S10 ). Kit Wsh/Wsh mice spontaneously show elevated levels of neutrophils in their spleens [35] ; however, we confirmed that the neutrophil levels were the same as those in the colons of Kit +/+ , Kit Wsh/+ and Kit Wsh/Wsh mice under naïve conditions ( Fig. 1h,i ). To exclude the possible involvement of other immunological defects in Kit Wsh/Wsh mice, such as the involvement of the Corin gene, which is associated with type II transmembrane serine protease [35] , we further confirmed the amelioration of intestinal inflammation in conditional MC-deficient mice ( Fig. 2d–h ). These findings strongly suggest that P2X7 on MCs has a pivotal role in the development of murine and human intestinal inflammation. P2X7 purinoceptors are expressed on T cells, DCs, macrophages and ECs [9] , [10] , [11] , [25] , [36] . In a recent study, ATP/P2X7-mediated signalling inhibited the generation and function of regulatory T cells and ATP stimulation led to their conversion into Th17 cells via an IL-6-dependent pathway; thus, the P2X7 antagonist OxATP inhibited colitis [37] . In that study, ATP/P2X7-mediated regulation of regulatory T cells was involved in the chronic phase of intestinal inflammation, which takes about 4 weeks for disease development [37] . Similarly, ATP-mediated DC activation occurs in the chronic phase of intestinal inflammation through the preferential induction of Th17 cells, although whether this is mediated by P2X7 remains to be seen [38] . In contrast, ATP/P2X7-mediated MC activation in our model was important in the development of T-cell-independent acute colitis, which occurs within 1 week. Thus, our study and those of others [37] , [38] complement each other by reflecting the complicated pathological aspects and kinetics of the acute and chronic phases of intestinal inflammation mediated by ATP and P2X7. We also found that the expression level of P2X7 receptors differed depending on the tissue and animal species. First, colonic MCs expressed high levels of P2X7, but skin MCs did not ( Fig. 3a ). Second, in contrast to MCs, some macrophages (for example, microglia and RAW264.7 cells) expressed higher levels of P2X7 than did colonic macrophages ( Fig. 3b and data not shown). Third, among the several types of immunocompetent cell in the colon, MCs expressed the highest levels of P2X7 ( Fig. 3a,b ). Fourth, we found P2X7 expression on human colonic ECs, but not on murine colonic ECs ( Figs 3b and 5g ). In addition, as reported previously [36] , P2X7 expression on ECs was downregulated in the colons of CD patients; instead, CD patients showed increased numbers of P2X7 + MCs in their colons ( Fig. 5g,h ). It is important to note that, like murine MCs, human lung MCs express functional P2X7 (ref. 39 ). Therefore, although we must recognize the similarities and differences between mouse and human intestinal inflammation and MC distribution, ATP/P2X7-mediated MC activation seems to have a major role in the development of intestinal inflammation. We found elevated levels of extracellular ATP in the colons of TNBS-treated mice ( Fig. 6a ). This high ATP concentration was most likely achieved by a combination or cascade of several ATP production pathways (for example, cell injury or lysis [7] , pattern recognition receptor-mediated activation of monocytes [40] and commensal bacteria [38] ). In our tissue culture system, we detected elevated release of ATP (40 μM) in the inflamed colon compared with the control ( Fig. 6 ); however, at least 100 μM ATP was required for MC activation in vitro in the single cell culture system ( Fig. 7b ). This disparity likely reflects the differences in the culture conditions. Unlike in the single cell culture system, the concentration of secreted ATP in the tissue culture system could have been diluted in the culture medium, or ATP could have been consumed rapidly by activated inflammatory cells in the tissue. Alternatively, a lack of commensal bacteria-derived ATP in the tissue culture system as a result of the inclusion of antibiotics may have reduced the ATP level. Another possibility is that the abundant endogenous ATP-degrading enzymes (for example, CD39) in the colon tissue may have degraded some of the ATP. In support of this idea, a suppressive role for CD39 in intestinal inflammation has been reported [41] . We found that ADP-reactive P2Y1 and P2Y12 receptors were expressed on colonic MCs ( Fig. 7c ), but inhibition or knockdown of these receptors did not suppress the CD63 expression ( Fig. 7d,e ; Supplementary Fig. S8a ). In previous studies, stimulation of MCs with ADP (0.05–50 μM) has led to calcium influx via the P2Y1- but not the P2Y12-mediated pathway [42] , whereas our results indicate that CD63 expression required a higher concentration of ADP and was not suppressed by a P2Y1 inhibitor ( Fig. 7b,d ). This finding indicates that P2Y purinoceptors are not involved in the induction of CD63 + -activated MCs that is mediated by high concentrations of ADP. However, we found that adenylate kinase and ATP synthase converted ADP back to ATP, which subsequently induced P2X7 purinoceptor-dependent MC activation. A similar conversion of ADP to ATP has been reported for endothelial cells [27] . Among adenylate kinases, AK2 was highly expressed on MCs and had a pivotal role in the conversion of ADP to ATP ( Supplementary Fig. S9a,b ). As another P2Y ligand (UTP) did not induce MC activation ( Fig. 7b ), our findings suggest that ADP could be converted into ATP by AK2 and ATP synthase, and that this ATP subsequently activates MCs through P2X7 purinoceptors. In addition, colonic MCs do not express ecto-5′-nucleotidase (CD73), an enzyme that degrades ADP into adenosine, which has anti-inflammatory effects in intestinal inflammation [43] . Therefore, our study indicates that MCs express CD39, adenylate kinases and ATP synthase, but not CD73, to preferentially convert ADP to ATP for the exacerbation of inflammatory responses through P2X7 purinoceptors. Here, we showed that colitis aggravated by P2X7-mediated activation of MCs was independent of the inflammasome pathway, and that P2X7-mediated activation of MCs promoted TNFα production by effector cells to further promote intestinal inflammation [44] . Our findings also suggest that MCs exacerbate inflammation by recruiting neutrophils to produce abundant TNFα, but less IL-10 than is produced by other cells (for example, eosinophils, DCs and macrophages; Supplementary Fig. S10d ). This neutrophil recruitment was mediated by the production of IL-1β, LTs and chemokines, which are potential targets for the treatment of colitis. Mice with experimentally induced colitis that lack CXCR2 or 5-LO (a key enzyme for converting arachidonic acid to LTs), as well as mice treated with inhibitors of CCR2, CXCR2 or 5-LO, show reduced inflammation and less neutrophil recruitment in their colons [33] , [45] , [46] . Moreover, given that ATP promotes neutrophil migration [47] , it is possible that P2X7-dependent LT and chemokine production, as well as ATP generation via AK2 and ATP synthase from MCs, could amplify neutrophil infiltration of the colon. These data collectively indicate that MCs are key factors in the induction of intestinal inflammation and also recruit neutrophils to heighten inflammatory responses. P2X7-dependent MC activation could, therefore, be a target for the treatment of intestinal inflammation. Mice and human samples Female C57BL/6 mice were purchased from CLEA Japan. Rag1 −/− and P2x7 −/− mice were obtained from Jackson Laboratory (Bar Harbour, ME, USA). MC-deficient Kit W-sh/W-sh mice were obtained from Dr H. Suto (Atopy Research Center, Juntendo University, Japan). For the conditional MC-deficient analysis, Mas-TRECK tg mice were injected intraperitoneally with 250 ng of diphtheria toxin for 5 consecutive days and then with 150 ng every other day [18] . Caspase-1 −/− mice were backcrossed with C57BL/6 mice; F5 mice were used for this experiment [48] . All mice were maintained under specific-pathogen-free conditions at the Experimental Animal Facility of the Institute of Medical Science, the University of Tokyo. All experiments were approved by the Animal Care and Use Committee of the University of Tokyo. MC reconstitution was performed as described previously [49] . Briefly, BM-derived MCs were obtained from P2x7 +/+ , P2x7 −/− or caspase-1 −/− mice as described previously [22] . BM-derived MCs (5×10 6 ) were intravenously transferred to Kit W-sh/W-sh mice at two time points (0 and 14 days). The reconstituted mice were used 3 months after the last transfer. Colon specimens from UC and CD patients and healthy volunteers were obtained by endoscopic biopsy at Osaka University Hospital. All subjects provided written informed consent, and the study protocol was approved by the Ethics Committee of Osaka University Graduate School of Medicine (no. 08243) and the Institute of Medical Science, The University of Tokyo (no. 20-67-0331). Experimental colitis For TNBS-induced colitis, anaesthetized mice (18–22 g) were sensitized with 2.5% TNBS (Sigma-Aldrich) together with acetone and olive oil [50] . After 1 week, after a 3-h fast, the mice were given 100 μl of 2.5% TNBS in 50% ethanol via a flexible feeding tube that maintained their heads in a vertical position for 10 min. The control group received only 50% ethanol. Weight changes were recorded daily, and tissues were collected for histological analysis and isolation of mononuclear cells from the colonic lamina propria. For mAb treatment, mice were injected intraperitoneally with 0.5 mg of mAb (1F11 or an isotype control) 1 day before being given TNBS/EtOH intrarectally. mAb administration was continued for 3 days. For P2Y12 inhibition with clopidogrel sulphate, (Wako, Osaka, Japan), mice received clopidogrel (0.5 mg ml −1 ) in their drinking water from 3 days before intrarectal administration of TNBS/EtOH until the end of the study [50] . For DSS-induced colitis, mice were given 3.5% DSS (Wako, for C57BL/6) or 2.5% DSS (MP Biomedicals, Illkirch, France, for Mas-TRECK tg mice) in their drinking water for 5 days and their body weights were monitored daily [50] . In some experiments, non-hydrolysable ATP (adenosine 5′- O -(3-thio) triphosphate and O -(4-benzoyl)benzoyl adenosine 5′-triphosphate) or UDP-glucose (0.25 mg in 50% EtOH) was intrarectally administered and the effects were analysed 2 days later. In vitro MC stimulation and inhibition BM-derived MCs (2.5×10 5 ) were cultured with various concentrations of adenosine, ADP, ATP, UTP or anti-DNP-IgE with DNP-human serum albumin. Adenosine-3-phosphate 5-phosphosulfate (0.25 mM), carbenoxolone (10 μM), flufenamic acid (100 μM), pyridoxal-phosphate-6-azophenyl-2′,4′-disulfonate (100 μM), 4,4′-diisothiocyanatostilbene-2,2′-disulfonic acid disodium salt hydrate (100 μM), OxATP (0.5 mM), AD2P5 (1 mM), oligo (10 or 100 μM) or UDP (100 μM) was added to the cells for the inhibition assay [27] , [28] , [40] , [51] . All reagents were purchased from Sigma-Aldrich (St Louis, MO, USA, purity was ≥ 95%). 5-LO (BD Pharmingen, Franklin Lakes, NJ, USA) was stained after permeabilization with 0.2% Triton-X100 for 10 min; nuclei were stained with 4′,6-diamidino-2-phenyl indole. Cell preparation and flow cytometry ECs and lamina propria mononuclear cells were isolated from the colon, as described previously [52] . For flow cytometric analysis, cells were incubated with 5 μg ml −1 of an anti-CD16/32 antibody (10 μg ml −1 , Fc block, BD Pharmingen) for 5 min and stained for 30 min at 4 °C with fluorescence-labeled Abs specific for c-kit (0.2 μg ml −1 ), Gr-1 (0.4 μg ml −1 ), CD4 (1 μg ml −1 ), CD11b (0.2 μg ml −1 ), CD11c (0.4 μg ml −1 ), CD39 (0.4 μg ml −1 ), CD45 (0.4 μg ml −1 ), IgA (10 μg ml −1 ), B220 (0.4 μg ml −1 ; BD Pharmingen), CCR3 (2 μg ml −1 ), CXCR2 (4 μg ml −1 ; R&D Systems, Minneapolis, MN, USA), FcεRIα (0.4 μg ml −1 ), CD73 (0.4 μg ml −1 ), TLR2 (10 μg ml −1 ; eBioscience, San Diego, CA, USA), F4/80 (20 μg ml −1 ), CCR2 (10 μg ml −1 ), P2X7 (Hano43; 2 μg ml −1 ,Serotec, UK) or CCR1 (10 μg ml −1 , Abnova, Taiwan). Flow cytometric analysis and cell sorting were performed by using FACSCalibur and FACSAria (BD Biosciences, Franklin Lakes, NJ, USA), respectively. Sorted cells were stained with May-Giemsa stain in some experiments. Colonic MCs and BM-derived MCs were prepared as described elsewhere [22] . Establishment of an anti-P2X7 mAb (1F11) and an anti-CD63 mAb The procedure used to establish MC-specific mAbs is shown as a flowchart in Supplementary Figure S3 . Briefly, c-kit + FcεRIα + MCs were obtained as described previously [22] from the colons of mice that exhibited allergic diarrhoea. Purified colonic MCs (10 6 cells) were injected into the footpads of Sprague Dawley rats seven times, as described previously [53] . Lymphocytes were isolated from the spleen and inguinal lymph nodes and fused with P3X63-AG8.653 myeloma cells (CRL-1580; American Type Culture Collection, Manassas, VA, USA). The reactivity of each hybridoma to the colonic MCs was examined by means of flow cytometry. To identify antigens recognized by the mAbs, immunoprecipitation was performed with the mAbs, followed by Liquid chromatography–mass spectrometry analysis, as described previously [53] . Antigen specificity was confirmed by transfecting CHO cells with plasmids that encoded the murine P2X7 receptor and CD63. Measurements of membrane permeability and inflammatory mediators To assess membrane permeability, BM-derived MCs were washed twice with phosphate-buffered saline (PBS) and incubated with 1 mg ml −1 Lucifer yellow (Sigma-Aldrich) containing 250 μM sulfinpyrazone (Sigma-Aldrich). The MCs were then stimulated with 0.5 mM ATP (Sigma-Aldrich) for 15 min, as described elsewhere [12] . In the inhibition assay, 1 or 10 μg ml −1 of 1F11 mAb or the control antibody (Rat IgG2b) was added before ATP stimulation. The fluorescence signal of Lucifer yellow was determined by using fluorescence microscopy (BZ9000, Keyence, Osaka, Japan) and flow cytometry. To measure the production of cytokines, chemokines and LTs from MCs, BM-derived MCs (2.5×10 5 ) were stimulated with 2.5 mM ATP for 30 min, after which the supernatants were collected. Chemokine and cytokine production was detected with an inflammatory cytokine kit (BD Pharmingen). For IL-1β measurement, BM-derived MCs from wild-type, P2x7 −/− and caspase-1 −/− mice were stimulated with 0.1 μg ml −1 of LPS for 4 h, followed by ADP or ATP stimulation. LT C4/D4/E4 production was detected by use of an enzyme-linked immunosorbent assay (GE Healthcare Bio-Science, NJ, USA). For ATP, cytokine and chemokine measurements from the colon tissue, the colon tissues were isolated from mice 2 days after intrarectal administration of TNBS. Released ATP was measured by culturing colon tissues at 100 mg of tissue per 100 μl of RPMI1640 medium for 3 h and using a luminescence ATP detection system (PerkinElmer, Norwalk, CT, USA). Immunoprecipitation and western blotting Cell lysates obtained from BM-derived MCs or CHO transfectants (mouse P2X7 variants a, c and d and flag-mP2X7s, cloned from C57BL/6 mice) were analysed by western blotting and immunoprecipitation with 1F11 mAb or the control Ab. Membranes were probed with an anti-flag and a polyclonal rabbit anti-P2X7 antibody (Sigma-Aldrich). Histology Colonic tissues were fixed in 4% paraformaldehyde and embedded in paraffin. Tissue sections (5 μm) were stained with haematoxylin and eosin solution, as described previously [22] . For the detection of MCs and P2X7 expression in human specimens, colonic tissue sections were stained with antibodies for MC tryptase and P2X7 purinoceptors (Alomone Laboratories, Jerusalem, Israel). shRNA plasmid construction and lentiviral transduction For the construction of shRNA expression lentivirus vector plasmids, a series of oligonucleotide pairs were synthesized, as listed below. Each oligo pair was annealed and cloned into pmU6 [54] . Each mU6-shRNA cassette was then subcloned into the ΔU3 sequence of the 3′-LTR of the lentivirus vector plasmid pLCG to generate pLCG-shCD63 (sense: 5′-TTTGATTCTTGCTGCATCAACATAGCTTCCTGTCACTATGTTGATGCAGCAAGAATCTTTTTTG-3′, antisense: 5′-AATTCAAAAAAGATTCTTGCTGCATCAACATAGTGACAGGAAGCTATGTTGATGCAGCAAGAAT-3′), pLCG-shP2Y12 (sense: 5′-TTTGATCTACTAATGATTCTAACTGCTTCCTGTCACAGTTAGAATCATTAGTAGATCTTTTTTG-3′, antisense: 5′-AATTCAAAAAAGATCTACTAATGATTCTAACTGTGACAGGAAGCAGTTAGAATCATTAGTAGAT-3′) and pLCG-shAK1 (sense: 5′-TTTGCGAGAAGATTGTACAGAAATGCTTCCTGTCACATTTCTGTACAATCTTCTCGCTTTTTTG-3′, antisense: 5′-AATTCAAAAAAGCGAGAAGATTGTACAGAAATGTGACAGGAAGCATTTCTGTACAATCTTCTCG-3′) and pLCG-shAK2 (sense: 5′-TTTTGGAGCTAATTGAGAAGAATTGCTTCCTGTCACAATTCTTCTCAATTAGCTCCATTTTTTG-3′, antisense: 5′-AATTCAAAAAATGGAGCTAATTGAGAAGAATTGTGACAGGAAGCAATTCTTCTCAATTAGCTCC-3′). To obtain lentivirus-encoding green fluorescent protein (as a reporter gene) and shRNA for CD63, 293FT cells (6×10 5 ) were transfected with pLP1, pLP2, pLP-VSVG and pLCG-shRNA by using Lipofectamine 2000 (Invitrogen, Carlsbad, CA, USA) as per the manufacturer's protocol (Invitrogen). After 24- and 48-h incubations, lentivirus-encoding shRNA was collected. BM-derived MCs (1×10 6 ) or MC/9 cells were transduced with shRNA expression lentivirus stock in the presence of 8 μg ml −1 Polybrene (Sigma-Aldrich) [55] . After 24 h, the cells were washed and green fluorescent protein-positive cells were sorted by FACSAria and used for subsequent experiments. Quantitative real-time–PCR Total RNA was prepared by using TRIzol (Invitrogen) and reverse transcribed by use of Superscript VILO (Invitrogen), as described. Quantitative reverse transcription–PCR was performed with the LightCycler 480 II (Roche, Mannheim, Germany) and the Universal Probe Library (Roche). Primer sequences are listed in Supplementary Table S1 . Statistical analysis Statistical analysis was performed by using the unpaired two-tailed Student's t -test and Welch's t -test. The data are presented as means±s.e.m. How to cite this article: Kurashima, Y. et al . Extracellular ATP mediates mast cell-dependent intestinal inflammation through P2X7 purinoceptors. Nat. Commun. 3:1034 doi: 10.1038/ncomms2023 (2012).